Timing of inorganic phosphate release modulates the catalytic activity of ATP-driven rotary motor protein F 1 -ATPase is a rotary motor protein driven by ATP hydrolysis. The rotary motion of F 1 -ATPase is tightly coupled to catalysis, in which the catalytic sites strictly obey the reaction sequences at the resolution of elementary reaction steps. This fine coordination of the reaction scheme is thought to be important to achieve extremely high chemomechanical coupling efficiency and reversibility, which is the prominent feature of F 1 -ATPase among molecular motor proteins. In this study, we intentionally change the reaction scheme by using single-molecule manipulation, and we examine the resulting effect on the rotary motion of F 1 -ATPase. When the sequence of the products released, that is, ADP and inorganic phosphate, is switched, we find that F 1 frequently stops rotating for a long time, which corresponds to inactivation of catalysis. This inactive state presents MgADP inhibition, and thus, we find that an improper reaction sequence of F 1 -ATPase catalysis induces MgADP inhibition. F 1 -ATPase (α 3 β 3 γδε), a catalytic sub-complex of F 0 F 1 -ATP synthase, is a rotary motor protein fuelled by ATP hydrolysis [1] , [2] , [3] . Three subunits (α 3 β 3 γ) function as the minimum component of the rotating system, where the α 3 β 3 unit forms a cylindrical stator and the γ rotor subunit penetrates the centre of the cylinder [4] . The catalytic sites for ATP hydrolysis are located on each interface between the α and β subunits, mainly on the β subunits, and the three β subunits are always in different catalytic states [4] . The interconversion of the catalytic states of β subunits, which induces their conformational transition, drives the rotation of the γ subunit [5] , [6] , [7] . The rotary motion of F 1 can be directly visualized by optical microscopy [8] , [9] , [10] . The unitary step size of the rotation of F 1 is 120°, and each step is coupled to a single turnover of ATP hydrolysis [11] . The 120° step is further divided into 80° and 40° sub-steps [12] , [13] . The 80° sub-step is triggered by ATP binding and ADP release, each of which occurs on different β subunits [14] . The 40° sub-step is triggered by ATP hydrolysis and release of inorganic phosphate (P i ), which also occurs on different β subunits [14] , [15] . The catalytic state of the β subunits is tightly coupled to the rotation of the γ subunit; thus, F 1 can synthesize ATP from ADP and P i when the γ subunit is forcibly rotated in the reverse direction [16] , [17] . Mechanically induced ATP synthesis is the physiological role of F 1 of F 0 F 1 -ATP synthase, in which F 0 , a proton-driven motor protein, compels F 1 to rotate in the reverse direction for ATP synthesis. This reversibility of chemomechanical coupling is the prominent feature of F 1 among other motor proteins. To achieve reversibility of chemomechanical coupling, fine coordination of the reaction sequence, which properly induces the conformational transition of β subunits, is required. To understand the fine coordination mechanism, extensive studies have been dedicated to unveiling the basic reaction scheme for the rotation and catalysis of F 1 , focusing on the catalytic turnover of individual β subunits ( Fig. 1a ). In this scheme, an individual β subunit binds to ATP when the γ subunit is oriented at a specific angle, and the binding angles for the individual β subunits differ by ±120°. Each β subunit hydrolyses the bound ATP into ADP and P i after γ rotates another 200° from the ATP-binding angle [18] . In addition, the produced ADP and P i are released from the catalytic site after additional 40° and 120° rotations, respectively [14] , [15] , [19] , [20] . When the γ subunit returns to the original angular position, the β subunit initiates the next round of catalysis by binding to a new ATP. Thus, the reaction sequences among the three β subunits are well coordinated at the resolution of elementary reaction steps, which contributes to the reversibility of the chemomechanical coupling on F 1 . 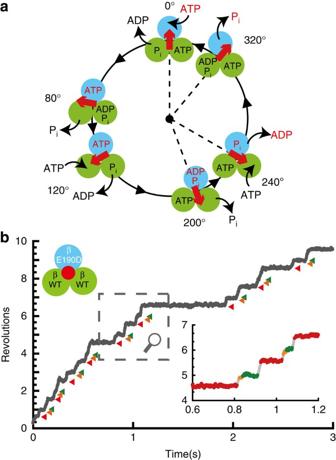Figure 1: Chemomechanical coupling scheme of F1-ATPase. (a) The circles and red arrows represent the catalytic state of the β subunits and the angular positions of the γ subunit. Each β subunit completes one turnover of ATP hydrolysis in a turn of the γ subunit, where the three β subunits vary in their catalytic phase by 120°. Regarding the catalytic state of the top β subunit (cyan), ATP binding, hydrolysis, ADP release and inorganic phosphate (Pi) release occur at 0°, 200°, 240° and 320°, respectively. (b) Time course of the rotation of the hybrid F1-ATPase, α3β(E190D) β2γ, in the presence of 1 mM ATP. Red, orange, and green represent the pause at 200°, 320°, and 360° for β(E190D), respectively. The inset shows a magnification of the time course. Figure 1: Chemomechanical coupling scheme of F 1 -ATPase. ( a ) The circles and red arrows represent the catalytic state of the β subunits and the angular positions of the γ subunit. Each β subunit completes one turnover of ATP hydrolysis in a turn of the γ subunit, where the three β subunits vary in their catalytic phase by 120°. Regarding the catalytic state of the top β subunit (cyan), ATP binding, hydrolysis, ADP release and inorganic phosphate (P i ) release occur at 0°, 200°, 240° and 320°, respectively. ( b ) Time course of the rotation of the hybrid F 1 -ATPase, α 3 β(E190D) β 2 γ, in the presence of 1 mM ATP. Red, orange, and green represent the pause at 200°, 320°, and 360° for β(E190D), respectively. The inset shows a magnification of the time course. Full size image Then, the question arises as to what happens when the reaction sequence of F 1 is changed. In the case of the hydrolysis step, although the timing of hydrolysis shifts by 80° relative to the authentic reaction angle, F 1 drives the rotation without interruption, demonstrating the robustness of the chemomechanical coupling of F 1 (ref. 21 ). In contrast, in the case of other elementary reaction steps, such as P i release, the effect of timing on rotary motion has not been examined so far, although we established a method to change the timing of P i release by using single-molecule manipulation [15] . In particular, the free energy change resulting from P i release was relatively high among reaction steps; that is, the rotary torque was mainly generated by P i release, and therefore, the effect of the timing of P i release on rotary motion is expected to be larger than that of other reaction steps [14] , [15] , [22] . In addition, the timing of P i release in F 1 is different from that in other motor proteins fuelled by ATP hydrolysis, such as kinesin and myosin, in which P i release occurs before ADP release [23] , [24] , and this difference is thought to be important for the reversibility of the chemomechanical coupling mechanism of F 1 (ref. 15 ). In this study, to further investigate the role of the finely coordinated reaction sequence of F 1 , we evaluate the effect of changing the timing of P i release on the chemomechanical coupling mechanism. When P i is released before ADP, we find that F 1 frequently stops rotating for a long time, which corresponds to inactivation of catalysis. This inactive state presents MgADP inhibition, and thus, we find that an improper timing of P i release induces MgADP inhibition. Rotation of hybrid F 1 We observed the rotation of hybrid F 1 carrying one β(E190D), that is, α 3 β 2 β(E190D)γ, in the presence of 1 mM ATP. Glu190 of the β subunit, the so-called ‘general base’, is known to be one of the most important residues for hydrolysis [25] , [26] , [27] , and its substitution into aspartic acid causes distinctively slow hydrolysis of ATP [28] and strong temperature sensitivity [29] . Therefore, the kinetic steps of the mutated catalytic site are easily distinguished from those of the other two sites. In the presence of 1 mM ATP, the hybrid F 1 showed three distinctive dwells caused by the incorporated β(E190D); the dwell for the temperature-sensitive reaction at 0° ( τ =32 ms) [15] , [29] , which is the same as the dwell at the ATP-binding angle, ATP hydrolysis at 200° ( τ =318 ms), and P i release at 320° ( τ =9 ms) (cyan in Fig. 1a,b ). The dwell time for P i release at 320° was prolonged because of the viscous drag of the rotary probe on γ as previously reported [30] , [31] . Hereafter, we refer to the angle for ATP hydrolysis by β(E190D) as the catalytic angle. Single-molecule manipulation to induce P i release During free rotation, one β hydrolyses ATP and another β releases the produced P i at the catalytic angle, resulting in a rotation of the γ subunit in an anticlockwise direction ( Fig. 1a ). In contrast to the free rotation, we recently succeeded in inducing the release of another produced P i from the same catalytic site used for ATP hydrolysis by arresting the γ subunit for a long time (>10 s) [15] , [22] . In this study, we used the same method to induce the release of produced P i immediately after ATP hydrolysis. For manipulation of γ rotation, a magnetic bead was attached to the γ subunit of F 1 , and the α 3 β 3 ring was immobilized on the glass surface. When the hybrid F 1 showed a pause for ATP hydrolysis by β(E190D) at 200°, we turned on the magnetic tweezers within ~450 ms ( Fig. 2a,b ) and arrested F 1 at ±10° from 200°. After a certain time period had elapsed, we turned off the magnetic tweezers and released F 1 from arrest. Then, F 1 roughly showed one of two behaviours without exception, as previously reported: rotating forward or restarting the hydrolysis-waiting pause ( Fig. 2a ). When F 1 shows the former behaviour, β(E190D) has already hydrolysed ATP and exerted a torque on the magnetic beads, whereas when β(E190D) shows the latter behaviour, it has not hydrolysed ATP because F 1 cannot generate torque unless β(E190D) catalyses hydrolysis. These behaviours are hereafter referred to as ‘on’ and ‘off’, respectively. Then, we measured the probability of the post-hydrolysis state as the probability of the ‘on’ case against the total number of trials, P ON . In the absence of P i in solution, P ON increased toward 100% as the arrest time increased; in contrast, in the presence of 100 mM P i , P ON did not change depending on the arrest time, which suggests that P ON depends on the time course of P i release from the catalytic site ( Fig. 2c ). 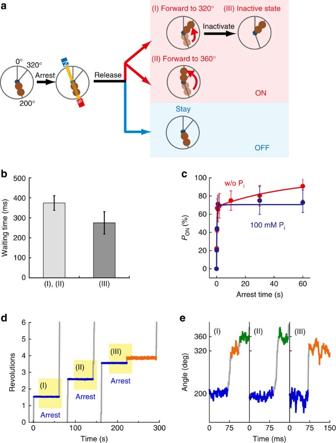Figure 2: Single-molecule manipulation for Pirelease. (a) Schematic representation of manipulation procedures. When the hybrid F1-ATPase paused at 200°; that is, the angle for ATP hydrolysis by β(E190D), we switched on the magnetic tweezers and arrested F1at ±10° from 200°. After release from arrest, F1-ATPase roughly showed two behaviours: rotating forward to next reaction angle (‘ON’), or staying at the original pausing angle (‘OFF’). In addition, the behaviour of ‘ON’ was classified into three types: (I) rotating forward to 320° and showing the distinctive pause for Pirelease (time constant (τ) is ~9 ms); (II) rotating forward to 360° (skip the pause at 320°); or (III) rotating forward to 320° and showing a long pause (τ=~39 s). (b) Hydrolysis-waiting time at 200° before F1-ATPase is arrested with the magnetic tweezers. The average waiting time was 370±37 ms for the behaviours (I) and (II) (light grey), and 275±56 ms for the behaviour (III) (grey). Error bars indicate s.d. (c) Time course ofPON. Red and blue points representPONin the absence or presence of 100 mM Pi, respectively. The number of arrest trials and molecules used for each data point were 23–108 and 8–19. The time courses were fitted with the reaction scheme; F1˙ATP↔˙F1(ADP+Pi)→F1˙ADP+Pi(solid lines). (d) Example of the time course of the arrest experiments (blue periods) corresponding to the behaviour of (I), (II) and (III), respectively. (e) Magnification ofd. Orange and green represent the pauses at 320° and 360°. Figure 2: Single-molecule manipulation for P i release. ( a ) Schematic representation of manipulation procedures. When the hybrid F 1 -ATPase paused at 200°; that is, the angle for ATP hydrolysis by β(E190D), we switched on the magnetic tweezers and arrested F 1 at ±10° from 200°. After release from arrest, F 1 -ATPase roughly showed two behaviours: rotating forward to next reaction angle (‘ON’), or staying at the original pausing angle (‘OFF’). In addition, the behaviour of ‘ON’ was classified into three types: (I) rotating forward to 320° and showing the distinctive pause for P i release (time constant ( τ ) is ~9 ms); (II) rotating forward to 360° (skip the pause at 320°); or (III) rotating forward to 320° and showing a long pause ( τ =~39 s). ( b ) Hydrolysis-waiting time at 200° before F 1 -ATPase is arrested with the magnetic tweezers. The average waiting time was 370±37 ms for the behaviours (I) and (II) (light grey), and 275±56 ms for the behaviour (III) (grey). Error bars indicate s.d. ( c ) Time course of P ON . Red and blue points represent P ON in the absence or presence of 100 mM P i , respectively. The number of arrest trials and molecules used for each data point were 23–108 and 8–19. The time courses were fitted with the reaction scheme; F 1 ˙ATP↔˙F 1 (ADP+P i )→F 1 ˙ADP+P i (solid lines). ( d ) Example of the time course of the arrest experiments (blue periods) corresponding to the behaviour of (I), (II) and (III), respectively. ( e ) Magnification of d . Orange and green represent the pauses at 320° and 360°. Full size image We extensively analysed the ‘on’ case and found that it can be classified into three behaviours; (I) rotating forward to 320°, (II) rotating forward to 360°; that is, skipping the pause at 320°, and (III) rotating forward to 320° and spontaneously stopping the rotation for a long time ( Fig. 2d,e ). When β(E190D) shows (I), it has hydrolysed ATP during its arrest but has not released the produced P i because the rate-limiting step at 320° is not hydrolysis by β(WT) but rather P i release by β(E190D) ( Fig. 1a ). F 1 cannot generate torque at 320° unless β(E190D) releases P i . When β(E190D) shows (II), it has hydrolysed ATP and simultaneously released the produced P i , and therefore, F 1 has already exerted torque for the step from 320° to 360° driven by P i release. Regarding the behaviour of (III), we have not identified the chemical state of β(E190D) thus far; however, the pausing angle is the same as that of the MgADP-inhibited state [32] . Hereafter, we characterize (III). First, we analysed the dwell time at 320° and calculated the probability of occurrence for each behaviour. As shown by the blue bars in Fig. 3a , distinctively long dwell times (longer than 100 ms), which correspond to the behaviour of (III), can be recognized. Then, we calculated the probability of occurrence of (III), that is , P III , as the number of events corresponding to the blue bars divided by total number of events in the histograms, and found that P III increased as the arrest time increased. As shown in Fig. 3b , we changed the time scale of the histogram to shorter bins (4 ms), and found that the histogram deviated from a single exponential decay model as the arrest time increased. For example, at 60 s of arrest, the first bin (<4 ms) contained many more events in which β(E190D) skipped the pause at 320° than expected from a single exponential decay that fit the data well after the first bin with a time constant of 9 ms (black line in Fig. 3b ), which was consistent with that of P i release in free rotation (rightmost panel in Fig. 3b ). Therefore, the first bin deviated from single exponential decay because of the behaviour of (II); accordingly, the first bin potentially includes behaviours of both (I) and (II). To calculate the probability of occurrence of (II), that is , P II , we fit the data points of the histograms (except for the first bin) to a single exponential curve with 9 ms as the time constant of P i release. P II was determined as the number of events that deviated from the single exponential curve in the first bin (green bars in Fig. 3b ) divided by total number of events of the histogram in Fig. 3a . In addition, we also calculated the probability of occurrence of (I), that is , P I , as the number of remaining events (light yellow bars in Fig. 3b ) divided by total number of events. 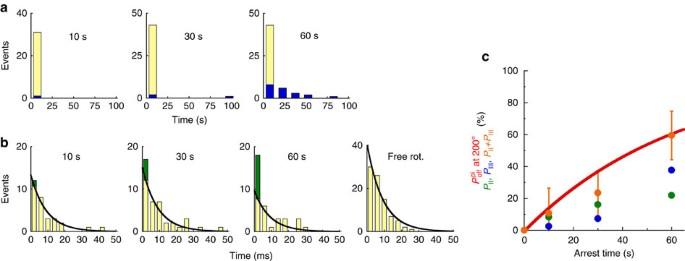Figure 3: Analysis of the effect of Pirelease at 200°. (a,b) Histograms of the dwell time at 320° after the release from 200° arrest for 10 s, 30 s, and 60 s, or during free rotation. The bin sizes of the histogram are 15 s foraand 4 ms forb. Blue bars inarepresent the number of pauses longer than 100 ms (behaviour (III)). The data after first bin inbwere well-fitted by the single exponential curve whereτ=9 ms (Pirelease dwell at 320°). The deviations of the first bins from the single exponential curves are coloured green (behaviour (II)). (c) Probability of Pirelease at 200°. The red solid line presents the simulation curve for Pirelease calculated from the analysis ofPONbased on the kinetic scheme as follows: F1·ATP↔ F1·(ADP+Pi)→F1·ADP+Pi. Green, blue and orange points represent the probability of occurrence of II (PII), III (PIII) and their sum (PII+PIII), respectively.PIIandPIIIwere determined from the analysis ofbanda, respectively. Figure 3: Analysis of the effect of P i release at 200°. ( a , b ) Histograms of the dwell time at 320° after the release from 200° arrest for 10 s, 30 s, and 60 s, or during free rotation. The bin sizes of the histogram are 15 s for a and 4 ms for b . Blue bars in a represent the number of pauses longer than 100 ms (behaviour (III)). The data after first bin in b were well-fitted by the single exponential curve where τ =9 ms (P i release dwell at 320°). The deviations of the first bins from the single exponential curves are coloured green (behaviour (II)). ( c ) Probability of P i release at 200°. The red solid line presents the simulation curve for P i release calculated from the analysis of P ON based on the kinetic scheme as follows: F 1 ·ATP↔ F 1 ·(ADP+P i )→F 1 ·ADP+P i . Green, blue and orange points represent the probability of occurrence of II ( P II ), III ( P III ) and their sum ( P II + P III ), respectively. P II and P III were determined from the analysis of b and a , respectively. Full size image Kinetic analysis of P i release and the inactive state From the analysis of P ON based on the irreversible reaction scheme ( Fig. 2c ) F 1 ·ATP↔ F 1 ·(ADP+P i )→F 1 ·ADP+P i , we can calculate the probability of P i release during arrest as P off Pi , as shown by the red line in Fig. 3c . For example, P off Pi is 37% and 60% for 30-s and 60-s arrest, respectively. Here, we compared P II and P off Pi , and found that P II was much smaller than P off Pi ( Fig. 3c , green). As mentioned above, we could not identify the chemical state of (III). Thus, we suspected that (III) was caused by P i release immediately after ATP hydrolysis and summed P II and P III . The sum of P II and P III was almost the same as P off Pi ( Fig. 3c , orange), suggesting that (III) was caused by P i release immediately after ATP hydrolysis. To confirm the relationship between (III) and P i release, we conducted the arrest measurement in the presence of high [P i ] (~100 mM), where P i did not affect the kinetics of ATP binding and produced ADP release [14] , [33] . When we added more than 10 mM P i in solution, P III was completely suppressed toward 0% ( Fig. 4a,b ), suggesting that (III) was induced after the P i release. Then, the kinetic scheme of (III) is given below (equation (1)), where, k hyd ATP , k syn ATP , k off Pi , k on Pi , and k a→i are the rate constants of ATP hydrolysis, synthesis, P i release, binding and inactivation of β(E190D), respectively. 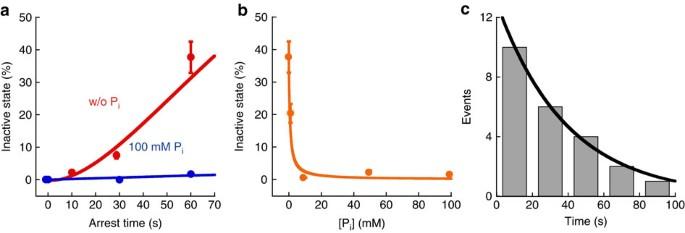Figure 4: Analysis of the long pause at 320°. (a) Time course ofPIIIin the absence (red) or presence of 100 mM Pi(blue). The red solid line is the fitting curve based on the kinetic scheme [1]. The blue solid line is the simulation curve based on the kinetic parameters determined from the fitting ofPIIIin the absence of Pi. (b) Relationship betweenPIIIfor 60 s arrest and Piconcentration. The simulation curve inFig. 4bwas redrawn against the Piconcentration. (c) Histogram of durations of the long pauses at 320° from the experiments of 10–60 s arrests. Solid line represents the fitting with single exponential curve where the time constant (τi→a) is 39 s. Bin size is 20 s. Figure 4: Analysis of the long pause at 320°. ( a ) Time course of P III in the absence (red) or presence of 100 mM P i (blue). The red solid line is the fitting curve based on the kinetic scheme [1]. The blue solid line is the simulation curve based on the kinetic parameters determined from the fitting of P III in the absence of P i . ( b ) Relationship between P III for 60 s arrest and P i concentration. The simulation curve in Fig. 4b was redrawn against the P i concentration. ( c ) Histogram of durations of the long pauses at 320° from the experiments of 10–60 s arrests. Solid line represents the fitting with single exponential curve where the time constant ( τ i→a ) is 39 s. Bin size is 20 s. Full size image As previously reported, k hyd ATP , k syn ATP , k off Pi , and k on Pi were given as 2.3 s −1 , 0.8 s −1 , 0.021 s −1 and 2 × 10 3 M −1 s −1 , respectively [15] . Then, from the fitting of P III in Fig. 4a based on the kinetic scheme as shown above, the only fitting parameter; k a→i , was determined as 0.019 s −1 . To verify this kinetic scheme, we fixed the arrest time as 60 s, and we re-plotted P III against P i concentration. Based on this kinetic scheme with the determined k a→i , we mathematically reproduced the experimental result of P III as shown in Fig. 4b . From these results, we confirmed that this inactive state was induced after P i release at 200° with a rate constant of 0.019 s −1 . We analysed the dwell time for activation from this inactive state ( Fig. 4c ). As shown in Fig. 4c , the histogram of the dwell time fit well to a single exponential curve, and we determined the time constant of activation, τ i→a , as 39 s, which was almost the same as that for activation from an MgADP-inhibited state [32] . In addition, the aforementioned phenomena in which the addition of a large amount of P i prohibited F 1 from lapsing into the inactive state ( Fig. 4a ) is a well-known feature of the MgADP-inhibited state [34] , suggesting that the inactive state revealed in this study corresponds to MgADP inhibition. MgADP inhibition, a common feature of F 1 -ATPase and ATP synthases from various sources [32] , [34] , [35] , [36] , [37] , is the catalytically inactive state. Although many biochemical studies have addressed MgADP inhibition, the mechanism of MgADP inhibition has remained elusive in the context of catalysis-rotation scheme. Here, we propose a simple model for how F 1 lapses into the MgADP-inhibited state during catalysis ( Fig. 5 ). We assume that the fundamental principle of MgADP inhibition is the loss of the driving energy of rotation derived from P i release. Our experimental data indicate that F 1 can continue rotating even if it releases P i before ADP at 200°, suggesting that F 1 principally stores the driving energy derived from P i release in conformation for 320°–360° rotation (grey solid line in Fig. 5 ). However, with a time constant of 0.019 s −1 , F 1 dissipates the stored energy during rotation before reaching 320° and lapses into MgADP inhibition at 320° (grey dash line in Fig. 5 ). The driving force of 320–360° rotation after inhibition is a thermal agitation, as our previous work suggests that thermally agitated rotation of γ over 30° induced activation from the MgADP-inhibited state [37] . Thus, the MgADP-inhibited state is so stable that it takes a long time to resume rotation, τ i→a =39 s ( Fig. 4c ) [32] . 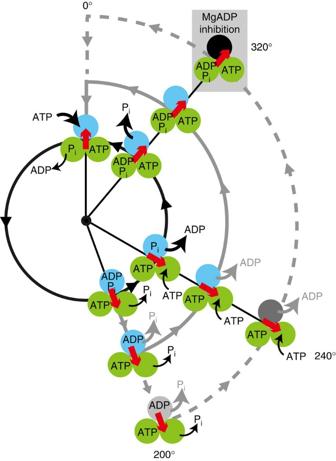Figure 5: Mechanism of MgADP-inhibited state. Black solid line: the normal reaction pathway of active F1-ATPase. F1-ATPase releases Piat 320°. Grey lines: alternative reaction pathways. F1-ATPase releases Pibefore ADP at 200°. F1-ATPase lapses into MgADP inhibition at 320° with some probability (dashed line). Figure 5: Mechanism of MgADP-inhibited state. Black solid line: the normal reaction pathway of active F 1 -ATPase. F 1 -ATPase releases P i at 320°. Grey lines: alternative reaction pathways. F 1 -ATPase releases P i before ADP at 200°. F 1 -ATPase lapses into MgADP inhibition at 320° with some probability (dashed line). Full size image The crystal structures co-crystallized with azide, including the original structure [4] , [38] , revealed that β at 320° (β E ) does not bind nucleotides or phosphate. Considering that azide is well known to stabilize the MgADP-inhibited state of F 1 , these structures demonstrate the structural features of the MgADP-inhibited state. Thus, it is highly probable that β in the 320° state of MgADP-inhibited F 1 has no bound nucleotide or phosphate, which is consistent with our model ( Fig. 5 ). It should be mentioned that the Walker group has challenged our reaction scheme of catalysis and rotation for active F 1 , on which the present work is based, that is, where P i is released from β in 320° state. Based on the recent crystal structure of MF 1 in which β in the 320° state is bound to Mg-free ADP [39] , they proposed that Mg and P i are released before ADP. Although the reason for this apparent discrepancy is not clear, it should be noted that most of the crystal structures solved so far had no bound nucleotide on β in the 320° state; the only exceptions are the above-mentioned structure [39] and a structure in a different study [40] . In addition, there are several experimental differences between the present study and the crystal structure study such as the species from which F 1 is derived and the buffer contents. A precise correlation between the crystal structure and the reaction model based on single-molecule experiments remains to be established. In vivo , F 1 forms F 0 F 1 -ATP synthase and synthesizes ATP by coupling with a rotary motion driven by F 0 . Previous studies revealed that MgADP inhibition suppresses ATP hydrolysis but not synthesis [41] . Recently, the rotary motion of the F 0 F 1 complex coupled to the synthesis of ATP was visualized at the single-molecule level [42] , [43] , [44] . For further understanding of the effect of MgADP inhibition on ATP synthesis, verification by single-molecule measurement of the F 0 F 1 complex is desirable in the future. Rotation assay To visualize the rotation of hybrid F 1 , α 3 β(E190D) β 2 γ, the stator region (α 3 β(E190D)β 2 ) was fixed on the glass surface, and a magnetic bead ( φ =0.3 μm; Seradyn, USA) was attached to the rotor part (γ) as a probe for rotation and manipulation. The experimental procedure was as follows. The flow chamber was constructed from an uncoated top coverslip and a bottom coverslip whose surface was modified with Ni 2+ NTA. F 1 solution, which was diluted in buffer A (50 mM MOPS-KOH, 50 mM KCl and 5 mM MgCl 2 , pH 7.0) to a final concentration of 200 pM, was infused into the flow chamber. After 5 min, unbound F 1 molecules were washed out with buffer A containing 10% bovine serum albumin, and then streptavidin-coated magnetic beads in buffer A were infused. After 10 min, unbound beads were washed out with buffer A. Finally, buffer A was infused with the indicated amount of ATP or P i . The rotating beads were observed under a phase-contrast microscope (IX-70 or IX-71; Olympus, Japan) with a × 100 objective lens. The rotation assay was performed at 23 °C. Manipulation with magnetic tweezers The stage of the microscope was equipped with magnetic tweezers that were controlled using custom-made software (Celery, Library, Japan). The rotary motion of the bead was recorded at 30 and 3,000 frames per second, simultaneously (FC300M, Takex, Japan; FASTCAM 1024PCI-SE, Photron, Japan). Images were stored in the hard disk drive of a computer as an AVI file and analysed using custom-made software. From the recorded images at 3,000 frames per second, we judged whether the operations precisely arrested the γ subunit at the targeted angle or not. How to cite this article: Watanabe, R. et al. Timing of inorganic phosphate release modulates the catalytic activity of ATP-driven rotary motor protein. Nat. Commun. 5:3486 doi: 10.1038/ncomms4486 (2014).